Stable prenucleation mineral clusters are liquid-like ionic polymers Calcium carbonate is an abundant substance that can be created in several mineral forms by the reaction of dissolved carbon dioxide in water with calcium ions. Through biomineralization, organisms can harness and control this process to form various functional materials that can act as anything from shells through to lenses. The early stages of calcium carbonate formation have recently attracted attention as stable prenucleation clusters have been observed, contrary to classical models. Here we show, using computer simulations combined with the analysis of experimental data, that these mineral clusters are made of an ionic polymer, composed of alternating calcium and carbonate ions, with a dynamic topology consisting of chains, branches and rings. The existence of a disordered, flexible and strongly hydrated precursor provides a basis for explaining the formation of other liquid-like amorphous states of calcium carbonate, in addition to the non-classical behaviour during growth of amorphous calcium carbonate. Calcium carbonate is a ubiquitous mineral, often created as a result of biomineralization, that is used by nature to perform many diverse functions in marine organisms, from skeletons and shells [1] to even optical devices [2] . It also represents a common scale forming from hard water leading to technological problems [3] , though deposition of carbonates can be put to beneficial use as a means of sequestering carbon dioxide [4] . Despite its economic, ecological and scientific relevance, our knowledge is far from complete in regard to the early stages of the complex process that can ultimately produce this mineral. Recently, there have been several key advances in our understanding of the nucleation and growth of calcium carbonate. It has been established that formation of amorphous calcium carbonate (ACC) and its subsequent transformation into crystalline phases provides a competing pathway to direct creation of the minerals calcite, aragonite and vaterite [5] , [6] , [7] . There is growing evidence that organisms exploit this alternative route for biomineralization as the amorphous phase can be stored until needed, at which point crystallization can be directed to yield the required crystalline polymorph. Furthermore, this process may not follow a conventional mechanism of the type envisaged within classical nucleation theory, in which an activation barrier must be overcome before significant association of ions can occur beyond simple ion pairing. The existence of stable prenucleation clusters of calcium carbonate before nucleation was initially shown by ion potential measurements in combination with analytical ultracentrifugation [8] , and later confirmed by cryogenic transmission electron microscopy [9] . The size of these clusters has been estimated to be either ~2 nm or 0.6–1.1 nm from the two experimental techniques, respectively; the discrepancy may be explained depending on the differing sensitivity of the methods to the surrounding hydration layer. While evidence grows for the presence of such stable clusters, the nature of these species in terms of composition and structure remains 'open to speculation' [10] . Following the above experimental work, there have been attempts to use computer simulation to understand the formation of ACC [11] . Based on a force field model that was accurately calibrated against experimental free energies of solvation [12] , we have previously shown that both the free energy of ACC should monotonically decrease as more ion pairs of calcium carbonate add from solution and that the initial association of ion pairs also lowers the free energy, suggesting that nucleation of this material may be barrierless and therefore completely non-classical [13] . This finding unfortunately appears to contradict experiment. These earlier simulations were for solutions of pure calcium (Ca 2+ ) and carbonate (CO 3 2− ) ions, that is, at high pH, whereas at experimental conditions, the pH is lower and bicarbonate ions (HCO 3 − ) dominate the equilibrium. Experimental measurements of the drop in free calcium at the point of nucleation ( Δn ) show that the magnitude of this event decreases with increasing pH [8] , as shown in Supplementary Figure S1 , apparently consistent with the simulations in the limit of high pH. Despite the above investigations, the details of the prenucleation form of calcium carbonate remain unclear. The challenge is to conceive of a structural form that can exist with a stability intermediate between ion pairs in solution and the amorphous phase. Any such structure must retain a high degree of hydration otherwise its enthalpy would be less exothermic than that of the ion pairs, which are strongly solvated in water. Conversely, such clusters must also exhibit a high level of disorder to compete entropically with ACC. To resolve this issue, we have performed molecular dynamics simulations of ions in solution to probe the details of their association. While it would normally be highly improbable to observe significant levels of aggregation using unbiased simulations, in this case a direct approach is feasible due to the spontaneous nature of cluster formation. In general, both the concentration of ions and pH can influence the balance of equilibria in solution, and we have therefore explored their impact for the specific case of calcium carbonate. Concentrations between 0.5 and 0.06 M are explored using extensive simulations of up to 70 ns. Here, the lower bound is approximately an order of magnitude greater than the experimental values at which it is possible to maintain solutions containing prenucleation clusters without them undergoing nucleation. In order to make direct contact with the actual experimental conditions, we have also performed more limited simulations for systems containing up to 6.4 million atoms that allow the bicarbonate and calcium concentrations to be reduced to 10 and 0.4 mM, respectively. By varying the relative concentrations of carbonate and bicarbonate ions, we have also simulated pH values in the range of 8.5–11.5, thereby spanning the experimental conditions. In the present work, we show that the stable prenucleation clusters of calcium carbonate are in fact ionic polymers consisting of chains of cations and anions held together by only ionic interactions. These chains can be linear or branched, with a dynamic structure that is constantly evolving, yet stable with respect to the separated solvated ions. Atomistic simulation of speciation Starting from free ions in solution, the initial stages of speciation involve the expected formation of the ion pair, CaCO 3 0 , and to a lesser extent, CaHCO 3 + (ref [14] ). At the lower end of the pH range studied, where there is an excess of bicarbonate anions, further association is observed to form species of calcium coordinated to two or even three bicarbonate anions at 0.5 M, though bicarbonate ion pairing becomes unimportant as the concentration decreases. In contrast, calcium and carbonate begin to assemble themselves into a new structural motif consisting of chains of ions resembling a polymer ( Fig. 1 ). These clusters can also include bicarbonate ions at low pH, but normally only at the end of the chain. As time progresses these chains lengthen by further collisions with ion pairs and/or ions. 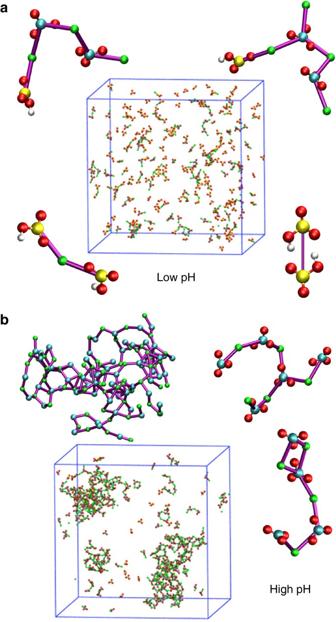Figure 1: Species observed in simulations of calcium (bi)carbonate solutions. (a,b) Illustration of the species observed at low and high pH, respectively, with snapshots of the simulation box for 0.5 M at the centre (animations of the time–evolution of the simulation are available asSupplementary Movies 1 & 2for pH 10 and 9.5, respectively). Here atoms are represented as spheres where calcium, carbon of carbonate, carbon of bicarbonate, oxygen and hydrogen are coloured green, blue, yellow, red and white, respectively. Ca–C and C–C distances below the cutoffs of 3.9 and 5.0 Å, respectively, are highlighted by purple bonds. For the largest cluster (top ofb), the oxygen atoms are omitted for clarity so that the connectivity is apparent. Figure 1: Species observed in simulations of calcium (bi)carbonate solutions. ( a , b ) Illustration of the species observed at low and high pH, respectively, with snapshots of the simulation box for 0.5 M at the centre (animations of the time–evolution of the simulation are available as Supplementary Movies 1 & 2 for pH 10 and 9.5, respectively). Here atoms are represented as spheres where calcium, carbon of carbonate, carbon of bicarbonate, oxygen and hydrogen are coloured green, blue, yellow, red and white, respectively. Ca–C and C–C distances below the cutoffs of 3.9 and 5.0 Å, respectively, are highlighted by purple bonds. For the largest cluster (top of b ), the oxygen atoms are omitted for clarity so that the connectivity is apparent. Full size image Where the above chains differ from a conventional organic polymer is in the dynamic nature of their structure. Being held together only by ionic interactions, the chains can frequently break and reform allowing them to explore a range of configurations involving linear chains, rings and branched structures ( Fig. 2 ). Full details of the coordination numbers of ions within clusters can be found in the Supplementary Figures S2–S7 , including as a function of concentration and pH. Here, we focus on the high concentration case of 0.5 M where the majority of carbonate ions are part of clusters instead of ion pairs. In this case, the most common coordination number of carbonate by calcium is 2, which is consistent with the chain-like model. The next most common coordination numbers are 1 and 3, corresponding to an ion at the end of the chain and a branching point, respectively. Higher coordination numbers, which are characteristic of crystalline or ACC, are rarely observed. By forming a chain, only two waters are removed from the solvation sphere per ion, thereby retaining much of the enthalpy of solvation. Furthermore, these clusters have a dynamic structure, which includes the ability to fold and coil like a polymer. This conformational freedom and the associated entropic contribution to the free energy is the key to the stability of these dynamic clusters. 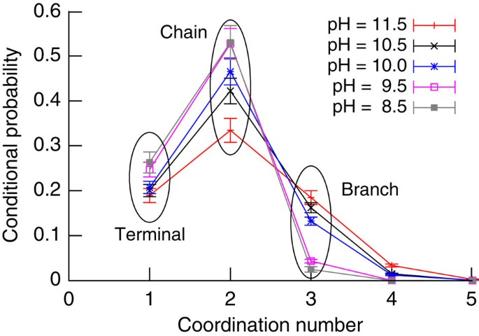Figure 2: Cluster coordination environment. Probability of finding a given coordination number of carbonate by calcium as a function of pH, conditional on the ion being part of a cluster. Points are labelled in the figure to indicate the underlying cluster structure corresponding to the coordination number. Here 'terminal' indicates a carbonate either at the end of a chain or in an ion pair; 'chain' represents a carbonate that bridges two calciums in a chain or ring; 'branch' denotes anions where the chain bifurcates. Error bars represent the s.d. of the average for successive 1-ns data windows. Figure 2: Cluster coordination environment. Probability of finding a given coordination number of carbonate by calcium as a function of pH, conditional on the ion being part of a cluster. Points are labelled in the figure to indicate the underlying cluster structure corresponding to the coordination number. Here 'terminal' indicates a carbonate either at the end of a chain or in an ion pair; 'chain' represents a carbonate that bridges two calciums in a chain or ring; 'branch' denotes anions where the chain bifurcates. Error bars represent the s.d. of the average for successive 1-ns data windows. Full size image Formation of chain-like structures is observed in all simulations, regardless of pH and composition. What varies with these conditions is the size distribution, the lifetime of a given length and the degree of branching along the chain. At low pH, the chain length is limited by competition between carbonate and bicarbonate, with the latter species generally acting as a chain terminator as it forms a weaker link between two calcium ions. At low concentration, growth is limited by the total number of ions available within the simulation cell. Furthermore, the growth of clusters becomes diffusion limited and so as the concentration decreases, the time taken to grow larger aggregates increases. The differing stability of clusters involving carbonate and bicarbonate can be determined from the cluster size distribution and its time evolution ( Fig. 3 and also Supplementary Fig. S8 for intermediate pH values). In the presence of excess HCO 3 − , an exponential decay in cluster size is observed. Here, the simulations are limited by the amount of carbonate and the timescale for species to encounter each other in the solution. For carbonate-rich systems, we find a size distribution with multiple peaks that shift to increasing values with time until a limiting size is reached at higher concentration. This indicates that the clusters we observe are stable, rather than metastable, with respect to solvated ions or ion pairs in solution. The limiting size reached in the simulations is a consequence of the number of ions present, whereas at lower concentrations the size would be limited by the balance between the frequency of collisions between ions and the cluster, versus the rate of ion loss. 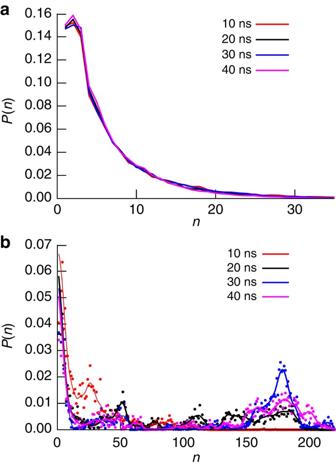Figure 3: Cluster size distribution. Probability,P(n), of finding a cluster containingnions averaged over successive time intervals of 10 ns for simulations at a calcium concentration of 0.5 M. Figures show probabilities for (a) pH 8.5 and (b) pH 11.5. Inb, dots represent the true data points while the lines represent smoothed fits to these values as a guide to the eye. Figure 3: Cluster size distribution. Probability, P ( n ), of finding a cluster containing n ions averaged over successive time intervals of 10 ns for simulations at a calcium concentration of 0.5 M. Figures show probabilities for ( a ) pH 8.5 and ( b ) pH 11.5. In b , dots represent the true data points while the lines represent smoothed fits to these values as a guide to the eye. Full size image Calcium coordination number Support for the above structural model of a chain-like structure comes from experiment ( Supplementary Table S1 ). By using a speciation model fitted to the experimental data it is possible to compute the average coordination number of calcium ions that are bound within stable prenucleation clusters. In the pH range of 9.25 to 10.0, we compute that this coordination number is 2±0.2 (average ± maximum deviation). Although this represents an average over the entire cluster, the only simple structural models that are consistent with this are a ring or long chain. Direct in situ structural information is difficult to obtain. However, ex situ EXAFS studies of rapidly quenched precursor species also point to twofold coordination of calcium by carbonate [15] . Furthermore, mass spectrometry indicates a series of clusters containing up to eight carbonate ions formed by successive ion pair additions [16] . Free energy sampling To quantify the thermodynamics of the polymer-like chains, we have computed the free energy as a function of the gyration radius of the calcium and carbon atoms, an approach similar to that used to understand the energetics of biomolecules [17] . 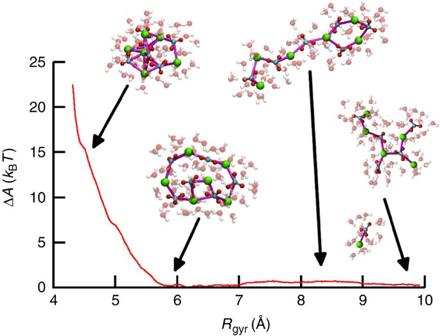Figure 4: Free energy as a function of radius for a six formula unit cluster. The Helmholtz free energy relative to the lowest energy structure,ΔA, is shown as a function of the radius of gyration,Rgyr, based on the calcium and carbon atoms. Here, the units of energy are Boltzmann's constant multiplied by temperature,kBT. Each atom has an ambient thermal energy of 1.5 in these units. Four sample atomic configurations are illustrated, along with their first solvation shell, for different radii to demonstrate the wide variety of structures accessible within ambient thermal energy in the case of the three largest radii. As can be seen from Figure 4 , where the free energy landscape for a six formula unit cluster is shown, this is very revealing. At small radii, corresponding to compressing the cluster towards a bulk-like structure, the free energy rises steeply. No stable state is found by compressing the radius alone, indicating that a significant activation barrier exists to dehydration. Outside of this, the free energy surface is incredibly flat and the radius of gyration can be changed by almost a factor of two at an energetic cost that is less than ambient thermal energy per degree of freedom. This remarkable flexibility is like distorting the shape of a liquid droplet. For this reason, we have named this stable cluster form of calcium carbonate dynamically ordered liquid-like oxyanion polymer (DOLLOP). We have deliberately not incorporated calcium carbonate into this name as we wish to stress that such species may also be observed for other oxyanions. Furthermore, given that Pouget et al . [9] have demonstrated that such clusters also exist after nucleation, in addition to being the first formed stable species, it seems inappropriate to continue using the phrase 'prenucleation clusters'. Figure 4: Free energy as a function of radius for a six formula unit cluster. The Helmholtz free energy relative to the lowest energy structure, ΔA , is shown as a function of the radius of gyration, R gyr , based on the calcium and carbon atoms. Here, the units of energy are Boltzmann's constant multiplied by temperature, k B T . Each atom has an ambient thermal energy of 1.5 in these units. Four sample atomic configurations are illustrated, along with their first solvation shell, for different radii to demonstrate the wide variety of structures accessible within ambient thermal energy in the case of the three largest radii. Full size image In an earlier simulation study [13] , it was found that the addition of calcium carbonate ion pairs to either small clusters of ion pairs (up to three formula units) or to both wet and dry ACC nanoparticles led to a very similar free energy profile. As all additions were exothermic, there was no evidence for a barrier to the growth of calcium carbonate from ion pairs into an amorphous phase. Here we have computed the radial free energy profile for a larger 36 formula unit piece of DOLLOP to compare against previous results for an amorphous nanoparticle of the same composition. This gives a similar radial free energy profile as that discussed above for six formula units of DOLLOP, though with a narrower radius range. Using data from previous simulations [13] , we can also determine the distribution of radii corresponding to ACC, both in its dry state and when containing structural water. 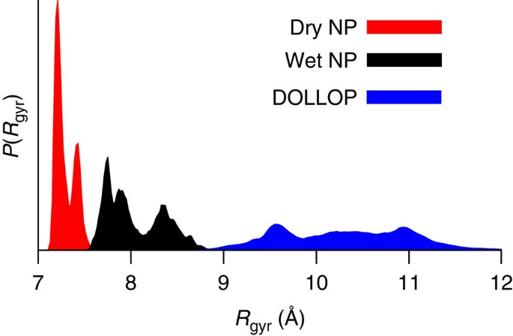Figure 5: Probability distributions as a function of radius of gyration. Probability distributions,P, are compared for dry and wet ACC nanoparticles (NP) containing 36 formula units of CaCO3, as well as for a DOLLOP cluster of the same size. The distributions for the NP are obtained by direct simulation, while that of DOLLOP comes from the free energy profile obtained by US. It should be noted that the total probability is unnormalized as the three regions come from separate simulations and cannot be collectively reweighted. From a comparison of the resulting radial probability distributions, shown in Figure 5 , it is clear that ACC and DOLLOP represent separate minima on the energy landscape. To compress the radius of DOLLOP towards that of the denser ACC nanoparticles it must undergo significant dehydration. Because of this, there must exist a significant activation barrier between DOLLOP and ACC that prevents spontaneous transitions from being observed between the two structures. The discrepancy between the findings of earlier simulations and experiment can therefore be resolved by the observation that DOLLOP and ACC have quite distinct densities and levels of hydration. Although the free energy profile for addition of a further ion pair to both cluster types is similar, it requires a nucleation event to occur for DOLLOP to transform to ACC. Figure 5: Probability distributions as a function of radius of gyration. Probability distributions, P , are compared for dry and wet ACC nanoparticles (NP) containing 36 formula units of CaCO 3 , as well as for a DOLLOP cluster of the same size. The distributions for the NP are obtained by direct simulation, while that of DOLLOP comes from the free energy profile obtained by US. It should be noted that the total probability is unnormalized as the three regions come from separate simulations and cannot be collectively reweighted. Full size image Speciation analysis of simulation data A speciation model has been fitted to the populations observed in the above models, allowing the equilibrium constants and corresponding free energies to be determined at 298.15 K. Here, we make the same assumption as used in the experimental analysis that the equilibrium constant for ion pair association is independent of cluster size, as supported by previous simulations [13] . Three separate fits were performed: (1) a fit to the data for pH 9.5, (2) a fit to the data for pH 10 and (3) a fit to the complete set of data points for all pH values simultaneously. The results are contained in Table 1 . Although the model contains some approximations (primarily that only the most numerous species are accounted for and not all possible reactions), three clear points emerge. First, the association of ion pairs to form larger clusters has an exothermic free energy. Second, the free energies obtained do not vary strongly with the pH of the system in the range examined. Third, the free energies obtained are close to those obtained from umbrella sampling (US) techniques thereby providing separate confirmation that the speciation model is valid. As the statistically best speciation data comes from high concentrations, the free energy values relate to these conditions. Table 1 Thermodynamics of speciation. Full size table To demonstrate the consequences of the free energies in Table 1 , we have computed the speciation at the experimental conditions, as given in Table 2 . Here, the fractions of calcium bound in ion pairs with both carbonate and bicarbonate are quoted, along with the fraction bound in larger clusters (DOLLOP). The calculations are performed at the same pH values considered experimentally with the same concentration of bicarbonate/carbonate buffer. A linear relationship is found between the amounts of added and bound calcium ions within the low concentration regime, in accord with the experimental findings. Therefore, we quote specific values only for one concentration value (0.4 mM) as an illustration. Table 2 Speciation of aqueous calcium carbonate/bicarbonate. Full size table The fraction of bound ions in Table 2 can be compared with the experimental values in Supplementary Table S1 . This shows that there is good agreement between the theoretical and experimental speciation, especially when considering the exponential dependence of the equilibrium constant on any error in the free energy. The largest discrepancy in the model is that the free energy of ion pairing between calcium bicarbonate is too exothermic by ~5 kJ mol −1 . To examine the influence of this, the experimental equilibrium constant for this reaction ( K bi ) of Plummer and Busenberg [18] can be substituted into the speciation model. Results for this scenario are also given in Table 2 . As can be seen, the effect of correcting this equilibrium constant is to greatly diminish the role of bicarbonate ion pairing to the point where it is negligible. Association of ionic species in solution has long been known for the case of ion pairs. Even the formation of triple ions is known to occur, for example between metal ions and the sulphate anion [19] . Beyond this, it is largely assumed that formation of higher oligomers corresponds to the creation of unstable species until the size of the critical nucleus is reached, after which the loss of translational entropy of the ions is compensated for by the cohesive energy of the proto-solid phase. Our results demonstrate that much larger stable chain-structured oligomers are possible for calcium carbonate. Unlike conventional organic polymers, these chains are held together by the ionic bond between a calcium cation and carbonate anion rather than a covalent linkage, something that is arguably unprecedented for this type of material. Hydrogen fluoride is known to form similar extended chains in both the gas/liquid phases and in ionic liquids [20] , [21] , but the weaker dipolar interactions between molecules are insufficient to preserve these oligomers in aqueous solution. Arguably a closer analogue to the present system is that of supramolecular polymers, where typically hydrogen bonds hold the fragments together, rather than covalent linkages [22] , [23] . The key to forming ionic polymers that are stable in solution is the balance between the solvation free energies of the cation/anion versus the strength of the cation–anion interaction. Given that other ions possess similar solvation properties to calcium and carbonate, there is no reason suppose that this phenomenon is unique to the present material. With any real or virtual experiment, it is important to discuss any potential limitations. In the present simulations every care has been taken to ensure that the thermodynamics of all interactions are calibrated against experiment and ab initio quantum mechanics where possible. However, no model for such complex systems can be perfect. To demonstrate that our observations are not an artefact of the underlying parameterization, we have also performed simulations with a different force field that includes reactivity [24] . Again the formation of flexible chains of ion pairs was found to occur, with the chains being, if anything, more stable than those observed with the present force field. Therefore the observation of stable dynamic chain-like structures is a robust finding, regardless of any small quantitative deviations that might exist. On a quantitative level, the finding that the free energy profiles for association of clusters involve differences at the level of ambient thermal energies is consistent with the experimental fraction of bound calcium being in the range 0.38 to 0.76. A driving force substantially greater than thermal energy, k B T , would lead to very different ratios of calcium concentration. The influence of concentration on the observations also deserves further discussion. Because of the limitations on what is feasible with current computers, it is only possible to obtain detailed statistical information from simulations at higher concentrations than those used in the experimental characterization of prenucleation clusters. To overcome this, a speciation model has been fitted to the simulation results at high concentrations. The equilibrium constants obtained can then be used to extrapolate to the lower concentrations employed experimentally. The theoretical speciation model is built on the assumption that DOLLOP grows by adding successive ion pairs with a constant exothermic free energy. At low concentrations, this yields an approximately linear relationship between the calcium added and the number of bound metal ions, which agrees almost quantitatively with the experimental observations, thereby supporting the validity of this extrapolation. A further argument relating to the influence of concentrations is that direct formation of a crystalline phase by a classical pathway may occur under the conditions simulated that bypasses the aggregation of ions to give stable DOLLOP clusters. As we are presently unable to simulate the nucleation event, we cannot comment definitively on what happens at this stage. However, it is possible to argue that prenucleation clusters of the type described are extremely likely to still exist. Under genuinely homogeneous conditions (that is, where there is no pre-existing seed or interface to grow from), ions have to assemble in solution before the nucleation of the crystalline phase. Previous simulations have already shown that calcite nanoparticles are only the most stable configuration beyond sizes of a few nanometres [13] . Hence, it is hard to explain why ions would form metastable ordered structures when there is a stable disordered configuration. From an entropic perspective, the direct creation of an ordered structure with a low volume in configuration space when there is an ensemble of structures with a large volume and lower free energy is improbable. The key point to emphasize here is that we make no claim that the present stable clusters described lie on all nucleation pathways that might occur under different conditions. However, they are very likely to be present during the early stages of speciation under most homogenous conditions, though either nucleation to ACC or dissolution and growth of a competing species may subsequently occur. Finally on the issue of concentration, we should consider the results obtained for the largest simulations, performed at the experimental conditions, in comparison with those conducted at higher concentrations. As simulations at this scale will be limited by the rate of diffusion and collision frequency of ions, it is not possible to observe the spontaneous formation of clusters in a statistically meaningful way. However, by placing clusters taken from simulations at higher concentrations into this simulation cell it is possible to determine whether there is any significant change in the structure and lifetime of the clusters at this lower concentration. As the timescale for water exchange in the calcium coordination environment is ~100 ps [25] , several nanoseconds of simulation is sufficient for a cluster to undergo a significant level of rearrangement and even dissociate completely if unstable. Four clusters containing four formula units of calcium carbonate were placed in the simulation cell so as to maximize the distance between them. 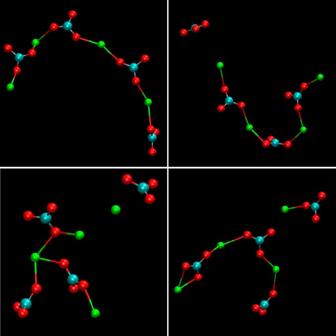Figure 6: Structures of the four formula unit prenucleation clusters. Structures shown represent the configurations of four separate clusters after 1 ns of simulation at experimental conditions ([Ca]=0.4 mM, [HCO3−]=10 mM, pH=10). Atoms are coloured green, blue and red for calcium, carbon and oxygen, respectively. Note that very similar structures can be seen in theSupplementary Movie 3where four ion pairs are started in a solvent-separated state in aqueous solution. Surrounding water and remote sodium, bicarbonate and carbonate species are omitted for clarity. During this simulation, the same variety of structures are explored as for simulations under different conditions; linear and branched chains are observed, while ions occasionally become solvent separated by one or more shells, though often return to the cluster again, as can be seen in Figure 6 . Hence, this behaviour is qualitatively no different from that observed for the same cluster either at high concentrations or when simulated in water alone ( Supplementary Movie 3 ). Changing the concentration alters the frequency of collisions between ions/ion pairs and clusters, and so the maximum size will vary according to the balance of association/dissociation events. Indeed, the lifetime of a particular cluster becomes longer, on average, as the concentration decreases due to the reduced frequency of collision. Despite this variation in cluster size and lifetime with conditions, the underlying structural characteristics of DOLLOP remain the same. Figure 6: Structures of the four formula unit prenucleation clusters. Structures shown represent the configurations of four separate clusters after 1 ns of simulation at experimental conditions ([Ca]=0.4 mM, [HCO 3 − ]=10 mM, pH=10). Atoms are coloured green, blue and red for calcium, carbon and oxygen, respectively. Note that very similar structures can be seen in the Supplementary Movie 3 where four ion pairs are started in a solvent-separated state in aqueous solution. Surrounding water and remote sodium, bicarbonate and carbonate species are omitted for clarity. Full size image In the process of biomineralization, organisms control the nucleation and growth of calcium carbonate to create complex-functional materials to serve a variety of purposes. While it still remains probable that much of this control is exerted through the ACC phase into which DOLLOP can ultimately transform by partial dehydration, there is also the possibility that this new form may also have a role under particular conditions. For example, it has been proposed [26] that certain peptides may bind chains of calcium carbonate, significantly altering the structure of the resulting material. Our work indicates that these chains are likely to be longer than the 3–4 ions previously speculated to exist as a cluster [26] , and is consistent with the observation of a long-range effect of the peptide. Other simulation studies have indicated that organic molecules (specifically those containing Asp residues in this case) can have a different influence by modifying the solvation environment of Ca 2+ even at a separation of ~4.9 Å [27] . Liquid-like phases of calcium carbonate have also been prepared by addition of acidic polypeptides to generate polymer-induced liquid precursor [28] . Recent work has demonstrated that liquid emulsions can be formed without the use of organic additives if the materials are levitated to prevent nucleation [16] , [29] , while addition of proteins can either stabilize or destabilize this liquid ACC [30] . The concept of a dynamic polymer structure involving highly hydrated calcium carbonate provides a unifying framework that connects all of these observations, while the existence of liquid precursors for materials beyond calcium carbonate indicates that this may well be a more general phenomenon. Finally, manipulation of this inorganic polymer offers new pathways by which organic molecules can influence biomineralization and biomimetic synthesis at the earliest stages of crystal growth [31] , [32] . Force field Here, existing parameters [13] for aqueous calcium carbonate systems were extended to include bicarbonate and sodium species. The intramolecular carbonate parameters were also refined to accurately describe the vibrational spectrum of this anion [33] , as described in Supplementary Table S2 , using the relaxed fitting algorithm within GULP [34] . As for carbonate, the water–bicarbonate parameters were fitted to the experimental free energy of solvation. Given there are limited experimental data to fit for bicarbonate, we have used quantum mechanical information to supplement this at the M06/6-31+G** to M06/6-311++G** level [35] in NWChem [36] . Quantum mechanical information is primarily used to fit repulsive interactions and to validate the energies/structures of complexes observed during molecular dynamics. Final parameters for bicarbonate inter- and intramolecular interactions are given in Supplementary Tables S3 and S4 , respectively. As association between calcium and carbonate/bicarbonate anions is an important feature of the speciation, we have computed the binding free energies of the ion pairs by US, yielding energies of −27 and −10.5 kJ mol −1 for CaCO 3 0 and CaHCO 3 + , respectively. When corrected to standard concentrations, these values are shifted to approximately −22 and −5.5 kJ mol −1 . The corresponding experimental values are −18 and −6.5 kJ mol −1 (ref. 18 ), though the value for CaCO 3 0 includes the contribution of prenucleation clusters. To model the experimental conditions, it is also necessary to include Na + whose interaction with carbonate was fitted to natrite (Lv/298 K) [37] under the approximations of full sodium occupancy and no modulation. The parameters were tested for eitelite [38] , with magnesium–carbonate parameters obtained from magnesite. Here, the largest error in the cell parameters was only 0.77%. The sodium–bicarbonate interactions were obtained by scaling the Buckingham A parameter for the carbonate case by the ratio of oxygen charges. These values were tested for sodium bicarbonate where errors in cell parameters were between 1.13 and 2.24%. Finally, the sodium–water interaction was taken from Grossfield et al . [39] and checked to ensure that the change of water model has negligible effect. Atomistic molecular dynamics simulation Molecular dynamics simulations were performed for solutions containing calcium, carbonate and bicarbonate ions under conditions of ambient temperature (300 K) and pressure (1 atmosphere). Concentrations of 0.5, 0.28 and 0.06 M were examined based on the molarity of the calcium ions, while the ratio of carbonate to bicarbonate was varied to yield conditions equivalent to pH values of 8.5, 9.5, 10, 10.5 and 11.5 based on the experimental equilibrium constant between the species. Cubic simulation cells were used of initial dimension ~10 nm that were varied within an NPT ensemble using a timestep of 1 fs. Typically this volume contains more than 30,000 water molecules. Single ions are initially distributed randomly throughout the solution while avoiding close contacts between atoms. All simulations were run for between 50 and 70 ns of real time using LAMMPS [40] . A chain of five Nosé–Hoover thermostats was employed with thermostat and barostat relaxation times of 0.1 and 1 ps, respectively. The electrostatics were treated using the Particle–Particle Particle–Mesh Ewald algorithm with a precision of 10 −4 . Additional simulations were performed using a larger cubic simulation cell of side ~40 nm, containing just over 2.1 million water molecules for a bicarbonate concentration of 10 mM and a carbonate/bicarbonate ratio consistent with a pH of 10. To match the experimental conditions just before the nucleation event at this pH, 16 Ca ions were placed in this cell to give a concentration of ~4×10 −4 M, while charge balance was maintained through the addition of sodium cations, as per the real system. Owing to the magnitude, these simulations were run for 1 ns. As simulations at this scale will be limited by the rate of diffusion and collision frequency of ions, it is not possible to observe the spontaneous formation of clusters. However, by placing clusters taken from simulations at higher concentrations into this simulation cell it is possible to determine whether there is any significant change in the structure and lifetime of the clusters at this lower concentration. US simulations [41] were performed using the PLUMED plug-in [42] in the NVT ensemble on a single cluster within a cubic cell containing ~6,300 water molecules (6 formula unit cluster) or 15,200 water molecules (36 formula unit cluster). Here, the radius of gyration was employed as the collective variable for US. The calculation for the 6 formula unit DOLLOP was performed with 16 windows, each run for 20 ns including equilibration, equally spaced in the interval 4.2–9.9 Å using a spring constant of 0.95 eV/Å. For the 36 formula unit case the interval spanned was 6.6–14.5 Å and the spring constant used was 0.5 eV/Å. The strength of each restraining potential was chosen so that the equilibrium probability distribution, P ( R gyr ), in each window overlapped with its neighbour at no more than 1.2 s.d. 's from the mean. Expansion by dissociation of the cluster was allowed, however, to suppress periodicity artefacts, the maximum distance between any two solute ions was prevented from exceeding half of the simulation cell by a smooth and continuous repulsive function. Probability distributions were computed only in regions where this repulsive function was negligible. The free energy was constructed using weighted histogram analysis within the WHAM software [43] . Analysis of simulation data Analysis of the unbiased speciation simulations is based on snapshots of the entire system taken at 5 ps intervals, and of the solute ions at intervals of 0.1 ps. The analysis of clustering was based on a geometric criterion for defining connections between ions. This required the distance connecting centres of two ions (taken as the coordinates of the carbon for molecular anions) to be shorter than 3.9 Å for Ca–C and 5.0 Å for C–C. These values were chosen to be close to the transition state separating directly coordinated species from those that are solvent separated. A recursive search over all connections was used to identify discrete instantaneous clusters. Cluster size statistics were accumulated over time windows of 1 ns to eliminate noise arising from sporadic ion–cluster and cluster–cluster proximity. Each cluster of non-trivial size was characterized by the number of ions with each coordination number in the range 1–5 (higher values not being observed). These quantities were averaged over the lifetime of the cluster. The cluster charge and composition were also recorded. Here, we adopted a more stringent cluster definition, requiring persistence with the same ions for >2 ps. Correspondingly, any cluster that breaks and re-forms within a time of 2 ps was considered to have persisted over that interval. Hence, the total number of ions assigned to these persistent clusters is a conserved quantity. At each frame we recorded the number and maximum size of both persistent and instantaneous clusters. We also recorded the number of ions of each type with zero connectivity, allowing direct connection to the experimental free ion concentration. The cluster size distribution information was used to perform a simple speciation analysis to provide a validation of the free energies for ion association. Here, we assume that equilibria exist between calcium and carbonate ions to form ion pairs, which are then able to associate further to form clusters with two separate equilibrium constants (that is, one for ion pairing and one for addition of an ion pair to a cluster). In the spirit of the experimental speciation model [8] , we assume that the equilibrium constant does not depend on the size of the cluster to which an ion pair adds. Recognizing the potential influence of bicarbonate ion pairing on the equilibria, we also include this as a competing process with a separate equilibrium constant. A least squares fit was then performed to the cluster populations obtained from the simulations. Experiment The experimental details are described elsewhere for potential measurements, titration and speciation [8] , as well as for structural analyses of quenched precursors [15] . In this work, data from these studies have been reanalysed and used for discussion. Specifically, the multiple-binding equilibrium introduced in previous work [8] has been examined in more depth. Evaluation of this physicochemical model gives the parameters, x and K , which are pH dependent. Here, x represents the number of binding sites for calcium ions on a carbonate ion, and the corresponding equilibrium constant is given by K . As shown by titration and calcium potential measurements [8] , equal amounts of calcium and carbonate ions are bound in prenucleation clusters. Hence, it is reasonable to assume that calcium ions have the same number of binding sites as carbonate ions, at the respective pH values. In solution, during the prenucleation stage, there are free ions and ions bound in clusters, and the number of binding sites is an averaged value that includes those ions with empty binding sites, that is, ions that are free in solution. In order to derive the macroscopic coordination number, N calcium , in prenucleation clusters from x , the fraction of bound ions, f , has to be taken into account; where n bound ( Ca 2+ ) and n free ( Ca 2+ ) are the amounts of bound and free calcium, respectively. N calcium , which is valid only for ions bound in clusters, is then given by: How to cite this article: Demichelis, R. et al . Stable prenucleation mineral clusters are liquid-like ionic polymers. Nat. Commun. 2:590 doi: 10.1038/ncomms1604 (2011).